Ferroelastic domain switching dynamics under electrical and mechanical excitations In thin film ferroelectric devices, switching of ferroelastic domains can significantly enhance electromechanical response. Previous studies have shown disagreement regarding the mobility or immobility of ferroelastic domain walls, indicating that switching behaviour strongly depends on specific microstructures in ferroelectric systems. Here we study the switching dynamics of individual ferroelastic domains in thin Pb(Zr 0.2 ,Ti 0.8 )O 3 films under electrical and mechanical excitations by using in situ transmission electron microscopy and phase-field modelling. We find that ferroelastic domains can be effectively and permanently stabilized by dislocations at the substrate interface while similar domains at free surfaces without pinning dislocations can be removed by either electric or stress fields. For both electrical and mechanical switching, ferroelastic switching is found to occur most readily at the highly active needle points in ferroelastic domains. Our results provide new insights into the understanding of polarization switching dynamics as well as the engineering of ferroelectric devices. Ferroelectric materials possessing a strong intrinsic coupling between the spontaneous polarization and strain are commonly chosen for use in piezoelectric sensors, mechanical switches and high-density non-volatile memories. For these materials, a long-standing, controversial question persists about the mobility of ferroelastic domain boundaries during ferroelectric switching [1] , [2] , [3] , [4] , [5] , [6] , [7] , [8] , [9] , [10] , [11] , [12] . Such boundaries separate regions where both the polarization vector and spontaneous strain change across the boundary. Several studies have found that these domain boundaries are highly mobile and significantly enhance the electromechanical response of the film [2] while other studies have conversely found that the lack of such switching hinders polarization reversal [9] , [13] . In tetragonal ferroelectrics, ferroelastic domain walls mediate a 90° rotation of the polarization vector and c axis of the unit, which necessarily produces local strains to accommodate the lattice parameter mismatch. First-principles calculations indicate the barrier to motion is much lower for these 90° domain walls than for 180° domain walls in PbTiO 3 that separate elastically equivalent domains [14] , but many experimental studies have shown 90° domain walls to be immobile in thin films [7] , [9] , [15] , [16] . This discrepancy has been found to be the result of substrate clamping and/or pinning by crystalline defects [17] , [18] such as dislocations, impurities or vacancies that interact with domain walls. Nevertheless, a few experimental studies suggested that the 90° domains (also known as a -domains, 90° domains possess polarization oriented in the plane of the film while c -domains possess polarization oriented out of the plane of the film) are mobile or switchable. For example, Kohli et al. [6] reported that the volume fraction of 90° domains could be reduced using external electric fields while Nagarajan et al. [2] found that mobility of 90° domain walls was enhanced in discrete patterned islands of Pb(Zr 0.2 Ti 0.8 )O 3 (PZT) thin films versus in continuous films. More recently, Ehara et al. [10] showed that ferroelastic domains in PZT thin films could move on a very short timescale on the order of hundreds of nanoseconds. Lee et al. [12] found that in a PZT capacitor the a -domains can split into fine a - and c -domain patterns during switching, resulting in the formation of 90° stripe domains. These varying experimental results suggest that the mobility of ferroelastic domain walls strongly depends on the specific system and the local environment, that is, the microstructure. This relationship between dynamic domain behaviour and microstructure remains unclear since it is difficult to extract these details from the large area aggregate responses measured with bulk techniques, such as X-ray diffraction or electrical characterization, or with surface probe techniques that provide limited subsurface microstructure information [2] , [6] , [7] , [8] , [9] , [10] , [15] . Recently developed in situ transmission electron microscopy (TEM) techniques, which enable switching behaviour to be correlated with specific microstructure and defects, provide a unique opportunity for domain dynamics studies [12] , [19] , [20] , [21] , [22] , [23] . Here we combine in situ TEM and phase-field modelling methods to study the nanoscale behaviour of individual ferroelastic domains under applied electric and stress fields in a thin Pb(Zr 0.2 Ti 0. 8)O 3 film. We find that the switching behaviour depends significantly on specific microstructures and that misfit dislocations play an important role in the mobility of ferroelastic domains. Ferroelastic domains located at the substrate interface in the film are stabilized by dislocations, which makes them difficult to remove, while similar domains at the free surface of the film, which are not associated with comparable dislocations, are not stabilized and thus are erased at moderate strength of either electric or stress fields. In both cases, ferroelastic domains that extend completely through the thin film were found to be much less mobile than their needle-shaped counterparts extending only partially through the thin film. The highly active tapered needle point of such partial ferroelastic domains observed in these films results from the inability of these regions to maintain a low-energy configuration of the polarization vectors (head-to-tail arrangement). Such active sites are the most mobile regions of ferroelastic domain walls for both electrical and mechanical switching. Our results provide new insights into polarization switching dynamics. Furthermore, the ability to control the polarization and strain by local ferroelastic domain switching provides a framework for exploiting multiple local microstructure-related parameters such as charge, lattice distortion and spin in strongly correlated materials. Electrical switching In this work, thin PZT films were subjected to in situ electrical and mechanical stimuli via a scanning probe depicted schematically in Fig. 1a . Films were grown on (001) SrTiO 3 or (110) DyScO 3 substrates with SrRuO 3 (SRO) buffer electrodes. Such films relax from a state of nominal compressive epitaxial strain through the formation of interfacial dislocation arrays. All films adopted a predominantly c axis-oriented mixed c / a / c -domain structure as shown in Fig. 1a,b . Analysis of the polarization [24] at ferroelastic domain boundaries via high-resolution high-angle annular dark field (HAADF) scanning TEM (STEM) images is shown in Fig. 1b , where the Pb sublattice offset is used to determine the polarization orientation in the film. The head-to-tail configuration at the 90° domain boundary minimizes the amount of bound charge at the domain wall [1] . Electric fields were applied parallel to the polarization in the c -domains, providing a driving force for the growth of the c -domains at the expense of unfavourably aligned a -domains. A typical chronological image series ( Fig. 1c ) shows that those a -domains clamped by interfaces are not mobile owing to effective interface clamping and/or dislocation pinning. At −18 V ( Fig. 1c ) no polarization switching of this a -domain is observed before dielectric breakdown in the film. The a -domain is eventually erased at –19 V, although this occurs during breakdown of the film and the formation of a damaged region proximate to the tip. 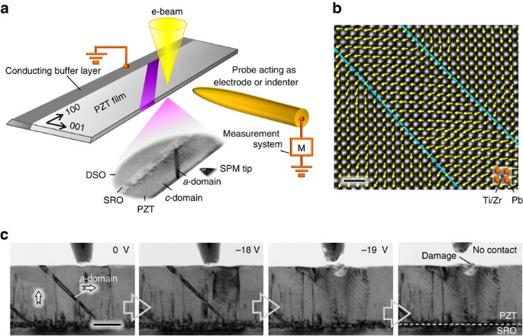Figure 1:Ferroelastic domain switching viain situTEM. (a) Schematic and TEM image of experimental set-up: a thin cross-sectional Pb(Zr0.2Ti0.8)O3film with a concentration of ferroelastic 90° domains (a-domains) was grown on SRO/DyScO3and SRO/SrTiO3. A mobile tungsten tip acts as one electrode for electrical switching with the SRO layer being grounded, whereas a diamond indenter is used for mechanical switching. (b) High-resolution HAADF STEM image ofc/a/c-domains overlaid with vectors describing the head-to-tail polarization arrangement. Scale bar, 1 nm. (c) Image sequence showing a clamped 90° domain is stable at applied negative voltages from 0→(−18) V. At −19 V, the domain is eventually erased and, simultaneously, damage to the film occurs due to the high strength of the electric field. Scale bar, 100 nm. Figure 1: Ferroelastic domain switching via in situ TEM. ( a ) Schematic and TEM image of experimental set-up: a thin cross-sectional Pb(Zr 0.2 Ti 0.8 )O 3 film with a concentration of ferroelastic 90° domains ( a -domains) was grown on SRO/DyScO 3 and SRO/SrTiO 3 . A mobile tungsten tip acts as one electrode for electrical switching with the SRO layer being grounded, whereas a diamond indenter is used for mechanical switching. ( b ) High-resolution HAADF STEM image of c / a / c -domains overlaid with vectors describing the head-to-tail polarization arrangement. Scale bar, 1 nm. ( c ) Image sequence showing a clamped 90° domain is stable at applied negative voltages from 0→(−18) V. At −19 V, the domain is eventually erased and, simultaneously, damage to the film occurs due to the high strength of the electric field. Scale bar, 100 nm. Full size image Generally, a -domains across the thickness of the film form nearly charge-neutral {101} 90° domain walls to achieve the most stable domain configuration in a tetragonal ferroelectric structure [14] . However, a -domains that do not extend through the thickness are also frequently observed in real samples, as shown in Fig. 2a , where a partial a -domain terminates in the middle of the film. Phase-field models of such partial domains indicated that they would not be stable in an ideal homogenous system, but instead are expected to switch back into a c -domain or extend all the way through the whole film, depending on the driving force determined by the competition between static electric energy and strain energy. Thus, these partial a -domains are likely stabilized by defects such as dislocations [18] , [25] , [26] . An atomic-resolution image in Fig. 2c shows a partial a -domain pinned by a pair of misfit dislocations with the Burgers vectors of near the bottom interface of the PZT thin film. In these samples, all partial a -domains located at the bottom interface were found to be stabilized and pinned by dislocations formed owing to the lattice mismatch between the epitaxially strained SRO electrode and the PZT film [18] , [25] . These a -domains adopt a needle-like shape [27] . The polarization map from this needle point ( Fig. 2e ) shows the domain boundary is no longer abrupt, in contrast to the conventional 90° domain walls shown in Fig. 1b , but the polar vectors seem to deviate from the regular polar axis ‹100› of the tetragonal phase of PZT, generating a transition zone where the in-plane polar state ( a -domain) transits gradually to the out-of-plane polar state ( c -domain). Owing to the inability to maintain a head-to-tail arrangement of the polarization vectors in this region, the domain needle point is both charged and relatively high in energy. This configuration makes partial a -domains effectively switchable, as shown in Fig. 2a . At −8 V, the partial a -domain begins to shorten as the polar vectors rotate 90° to coincide with the electric field. Switching begins from the needle tip, where the barrier to polarization rotation is lowest. With increasing bias, the partial a -domain gradually diminishes, shrinking along the long axis. However, the partial a -domain is never completely erased, even up to –30 V. Although the needle-like shape at the forward edge facilitates polarization rotation during the initial stages, the existence of large strains near the dislocations that is evidenced by both geometric phase analysis ( Fig. 2d ) and phase-field modelling locally stabilizes the in-plane polarization around the dislocation, as a unit cell is missing at each dislocation, and causes in-plane tensile strain that locally favours the a -domains, resulting in incomplete switching. The domain length is plotted as a function of time and is shown in Fig. 2b , and the change in length of the domain can be used to estimate the velocity of the domain wall during switching [28] . An inhomogenous distribution of the electric field resulting from the irregular geometry of the tip electrode and the built-in electric field [22] , however, makes it difficult to obtain a very precise estimate of the electric field-dependent velocity of the needle point. Besides non-uniform electric fields, various defect (for example, oxygen vacancies, dislocations)-induced pinning effects [22] , [28] may also account for the inhomogenous velocity during domain switching. After the external field is removed, the domain returns to its original length ( Fig. 2a ). 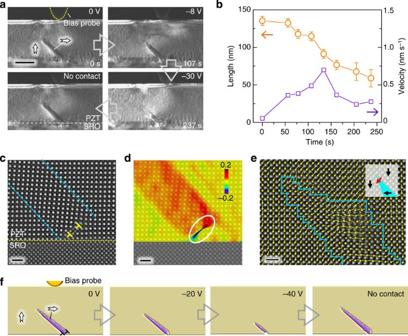Figure 2: Partial ferroelastic domain switching by electric fields. (a) Consecutive images showing bias-induced incomplete switching of a partial ferroelastic domain originating from the bottom interface as voltage is ramped from 0→(−30)→0 V. Rotation of the polarization during switching begins from the domain’s needle point. The partiala-domain cannot be erased completely even up to −30 V, and returns to its original extent after removal of contact. Scale bar, 100 nm. (b) The length and velocity (change in domain length with time) of the partial ferroelastic domain are plotted as functions of time. (c) High-resolution HAADF STEM image showing a partial ferroelastic domain is pinned by dislocations at the interface. Scale bar, 1 nm. The dislocation cores are labelled with ‘T’. 90° domain walls are highlighted by blue-dashed lines. (d) HAADF STEM image overlaid with in-plane strain colour map (strain tensorεxx(in-plane)) determined by geometric phase analysis showing huge local strain near dislocation cores (highlighted by white line). Scale bar, 1 nm. Colour scale for in-plane strain tensorεxx(in-plane): −0.2→0.2 nm/nm. (e) High-resolution HAADF STEM image of a ferroelastic domain’s needle point overlaid with polarization vectors showing the in-plane polar state (ina-domain) transitions gradually to the out-of-plane polar state (inc-domain), generating a highly active transition zone. Scale bar, 1 nm. The blue outline highlights the estimated domain boundary, which is not abrupt. The inset schematically shows the irregular polarization configuration at the needle point of the ferroelastic domain. (f) Phase-field modelling of electrical switching of a ferroelastic domain. A partial ferroelastic domain was stabilized in a poled [001] PZT film around two partial dislocations near the film interface. An electric potential was then applied to the surface of the film using an electrode modelled with a Lorentz-like function. In response to this potential, the extent of the ferroelastic domain in the system decreases. On removal of the applied potential, the ferroelastic domain returns to its original extent. Figure 2: Partial ferroelastic domain switching by electric fields. ( a ) Consecutive images showing bias-induced incomplete switching of a partial ferroelastic domain originating from the bottom interface as voltage is ramped from 0→(−30)→0 V. Rotation of the polarization during switching begins from the domain’s needle point. The partial a -domain cannot be erased completely even up to −30 V, and returns to its original extent after removal of contact. Scale bar, 100 nm. ( b ) The length and velocity (change in domain length with time) of the partial ferroelastic domain are plotted as functions of time. ( c ) High-resolution HAADF STEM image showing a partial ferroelastic domain is pinned by dislocations at the interface. Scale bar, 1 nm. The dislocation cores are labelled with ‘T’. 90° domain walls are highlighted by blue-dashed lines. ( d ) HAADF STEM image overlaid with in-plane strain colour map (strain tensor ε xx(in-plane) ) determined by geometric phase analysis showing huge local strain near dislocation cores (highlighted by white line). Scale bar, 1 nm. Colour scale for in-plane strain tensor ε xx(in-plane) : −0.2→0.2 nm/nm. ( e ) High-resolution HAADF STEM image of a ferroelastic domain’s needle point overlaid with polarization vectors showing the in-plane polar state (in a -domain) transitions gradually to the out-of-plane polar state (in c -domain), generating a highly active transition zone. Scale bar, 1 nm. The blue outline highlights the estimated domain boundary, which is not abrupt. The inset schematically shows the irregular polarization configuration at the needle point of the ferroelastic domain. ( f ) Phase-field modelling of electrical switching of a ferroelastic domain. A partial ferroelastic domain was stabilized in a poled [001] PZT film around two partial dislocations near the film interface. An electric potential was then applied to the surface of the film using an electrode modelled with a Lorentz-like function. In response to this potential, the extent of the ferroelastic domain in the system decreases. On removal of the applied potential, the ferroelastic domain returns to its original extent. Full size image The switching dynamics have also been simulated by phase-field modelling, as shown in Fig. 2f . A partial ferroelastic domain can be stabilized by two partial dislocations near the substrate interface with Burgers vectors of . In agreement with the experimental observations, application of an electric potential favouring out-of-plane polarization induces a reduction of the partial a -domain. Polarization near the dislocations, however, cannot be completely switched owing to the high elastic energy cost, even with large electric fields. After removal of the applied potential, the stabilized ferroelastic domain returns to its original extent. In contrast, partial a -domains originating at the free surface, rather than at the bottom interface, are not strongly pinned, more mobile and erased permanently with a moderate external electric field via 0→(−15)→0 V voltage ramps, as shown in Fig. 3a,b . Since ferroelastic domains usually inhibit the motion of 180° domain walls at low electric fields [9] , erasure of such ferroelastic domains should enhance the ferroelectric response in thin film devices [2] . Such a -domains, then, can be seen to be switchable between several metastable states and whether the domains exist as partial domains or extend completely through the film and whether the domain can be permanently switched to single c -domain is controlled by pinning defects. 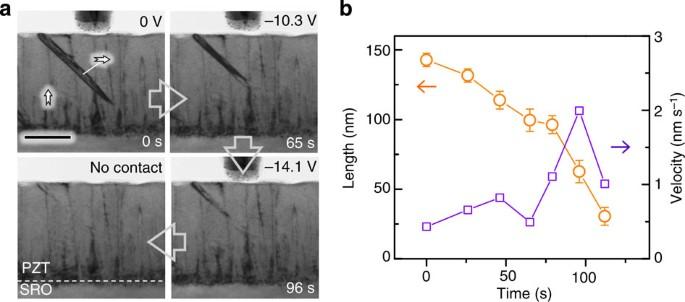Figure 3: Erasure of a partial ferroelastic domain by electric fields. (a) Consecutive images showing bias-induced erasure of a partial ferroelastic domain originating from the free surface. Scale bar, 100 nm. Note that the erasure occurs gradually as voltage is ramped from 0→(−15)→0 V. Rotation of polarization also starts from the domain’s needle tip. (b) The length and velocity (change in domain length with time) of the partial domain are plotted as functions of time. Figure 3: Erasure of a partial ferroelastic domain by electric fields. ( a ) Consecutive images showing bias-induced erasure of a partial ferroelastic domain originating from the free surface. Scale bar, 100 nm. Note that the erasure occurs gradually as voltage is ramped from 0→(−15)→0 V. Rotation of polarization also starts from the domain’s needle tip. ( b ) The length and velocity (change in domain length with time) of the partial domain are plotted as functions of time. Full size image Mechanical switching The mobility of ferroelastic domains under the application of a strain field was examined by using a nanoindenter to locally apply an in situ force to the PZT film. Similar to an electric field, strain can induce ferroelastic switching, since switching occurs when (ref. 29 ), where σ ij and ε ij are the stress and the strain tensors, E i and P i denote the magnitude of the electric field and polarization vectors, respectively, P s and E c are the spontaneous polarization and the coercive field, respectively, and Δ indicates the change between the initial and the post switching state. No electric field was applied, and the same PZT sample with a thin SRO buffer electrode was used. Application of a compressive force to the PZT thin film cross-section along the film normal favours the in-plane polarization, inducing the growth of a partial a -domain, which is shown in real time in the Supplementary Movie 1 and chronologically in Fig. 4a . The corresponding instantaneous load versus time and displacement curves are presented in Fig. 4b,c . 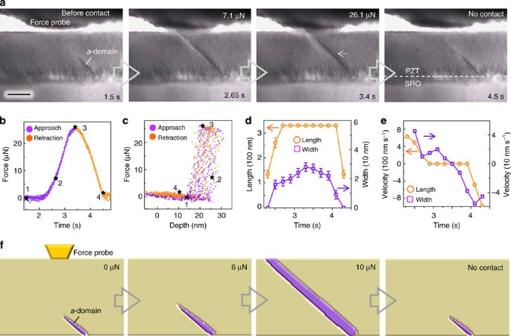Figure 4: Mechanical switching of a ferroelastic domain. (a) Bright-field still images extracted from a video showing the evolution of a partiala-domain during out-of-plane compression. The partiala-domain grows through the film thickness and widens at the surface of the film then returns to its original state after release of the stress. Scale bar, 100 nm. The corresponding load versus time curve (b) and load versus displacement curve (c). The purple points correspond to the approach branch and orange points correspond to the retraction branch. The highlighted black star points correspond to images ina. (d) The length and width of the ferroelastic domain are plotted as functions of time. The position for width measurement is highlighted by the white thin arrow ina. (e) The velocities of needle point motion and domain wall sideways movement (changes in domain length and width with time, respectively) are plotted as functions of time. (f) Phase-field modelling of mechanical switching of ferroelastic domain. Application of a force to a PZT film was modelled by assuming that the probe was a rigid indenter with size of 40 nm. As the applied load increases, the ferroelastic domain grows. With a large enough load, the ferroelastic domain extends to the film surface. On removal of the applied load, the domain returns to its original extent. Figure 4: Mechanical switching of a ferroelastic domain. ( a ) Bright-field still images extracted from a video showing the evolution of a partial a -domain during out-of-plane compression. The partial a -domain grows through the film thickness and widens at the surface of the film then returns to its original state after release of the stress. Scale bar, 100 nm. The corresponding load versus time curve ( b ) and load versus displacement curve ( c ). The purple points correspond to the approach branch and orange points correspond to the retraction branch. The highlighted black star points correspond to images in a . ( d ) The length and width of the ferroelastic domain are plotted as functions of time. The position for width measurement is highlighted by the white thin arrow in a . ( e ) The velocities of needle point motion and domain wall sideways movement (changes in domain length and width with time, respectively) are plotted as functions of time. ( f ) Phase-field modelling of mechanical switching of ferroelastic domain. Application of a force to a PZT film was modelled by assuming that the probe was a rigid indenter with size of 40 nm. As the applied load increases, the ferroelastic domain grows. With a large enough load, the ferroelastic domain extends to the film surface. On removal of the applied load, the domain returns to its original extent. Full size image Similar to electric switching, the polarization rotation driven by mechanical stress begins at the tapered needle point ( Supplementary Movie 1 ) of a partial a -domain. With increasing applied mechanical force up to 7.1 μN, the domain extends through the thickness to the surface along a roughly 45° orientation. This configuration allows the domain walls to adopt the typical lowest energy orientations parallel to {101} planes. Further increasing the force up to 26.1 μN widens the a -domain. Once the force is removed, the a -domain shrinks back to its original length, indicating the reversibility of the switching. The ferroelastic switching, then, appears completely reversible. While the distribution of stress in the test is not completely uniform because of irregular contact between the probe and the film, the maximum stress, p m , induced by the probe can be estimated from the Hertz contact model [30] : p m =3 F /2 πr 2 , where F is the force and r is the contact radius. Assuming a circular contact area and, given r =40 nm and F =7.1 μ N from Fig. 4a,b , the corresponding maximum stress is ~2.12 GPa. This value is well below the typical threshold for irreversible plastic damage for perovskite ferroelectrics [31] . Approach and retraction curves in Fig. 4c are nearly identical and indicate no mechanical damage occurred to the film during indentation. The domain length and width and the velocities of the needle point and domain wall sideways movements are plotted as functions of time and are shown in Fig. 4d,e , respectively. The velocity of the needle point in our experiments, ~100–1,000 nm s −1 , is nearly identical to the velocity of similar domains in bulk single-crystal LaAlO 3 at a moderate stress field [28] . However, the velocity of sideways movement of the domain walls, ~10–100 nm s −1 , is much lower than that of the needle point in our study. A previous study showed that in ferroelastic materials, needle domains can move even under small external forces and/or at low temperature while larger forces and/or at higher temperatures are required to cause additional sideways movement of domain walls [32] . These differences in velocity and threshold field between needle point motion and sideways movement are probably beacuse of the fact that the needle point has a high-energy domain front owing to the deviation from the regular polar axis in the polarization vector, as shown in Fig. 2e . Application of a force to a PZT thin film was also modelled with the phase-field method as shown in Fig. 4f . In agreement with the experimental results, the simulation shows that the partial a -domain grows and extends to the free surface under strain fields up to 10 μN. On reaching the film-free surface, the a -domain becomes wider, but returns to its original extent when the applied load is removed. Phase-field modelling was also used to study application of a force along the TEM-viewing direction of the sample (as schematically shown in Fig. 5a ), which cannot be easily studied with in situ TEM. In this simulation, the applied stress is assumed to uniformly increase the compressive strain in the viewing direction. The thin film sample, however, is assumed here to be laterally clamped, which prevents changes in the average in-plane strain in the system perpendicular to the viewing direction and corresponds to the application of a stress by an indenter much smaller than the in-plane length of the film and similar to the probe in the experimental set-up. Increasing the compressive strain along the viewing direction causes the partial a -domain to decrease in extent, as shown chronologically in Fig. 5b . During switching, the a -domain reduces in both length and lateral extent with increasing applied strain and, similar to the other switching cases, domain wall motion is fastest at the partial domain tip. On removal of the strain the domain returns to its original extent. 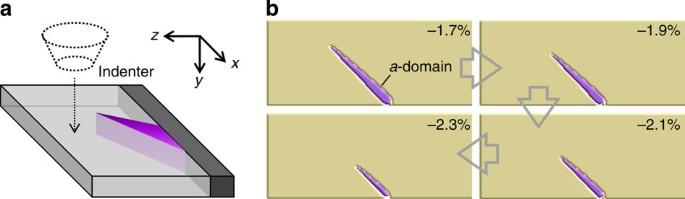Figure 5: Simulated response of clamped ferroelastic domain to applied strain along the zone axis. (a) Schematic showing application of a force along the viewing direction. (b) Application of the force was modelled as an increase in the strain along the TEM-viewing axis. This strain was added to the existing coherency strain of −1.7% along this direction. During the simulation, the average in-plane strain along thexdirection was held constant to model the clamped thin film. With increasing strain along the viewing direction (εyy) the extent of the ferroelastic domain is seen to become reduced, in contrast to a mechanical force applied to a clamped film along the thin film normal direction. However, the ferroelastic domain could not be completely removed from the thin film owing to the interfacial dislocations present at the substrate interface. Figure 5: Simulated response of clamped ferroelastic domain to applied strain along the zone axis. ( a ) Schematic showing application of a force along the viewing direction. ( b ) Application of the force was modelled as an increase in the strain along the TEM-viewing axis. This strain was added to the existing coherency strain of −1.7% along this direction. During the simulation, the average in-plane strain along the x direction was held constant to model the clamped thin film. With increasing strain along the viewing direction ( ε yy ) the extent of the ferroelastic domain is seen to become reduced, in contrast to a mechanical force applied to a clamped film along the thin film normal direction. However, the ferroelastic domain could not be completely removed from the thin film owing to the interfacial dislocations present at the substrate interface. Full size image Unlike mechanical switching with an out-of-plane mechanical force, both the c -domain and a -domain have identical in-plane strains along the TEM-viewing direction. Rather, switching occurs because of the stabilization of the c -domain by the strain state caused by both the applied strain and in-plane clamping of the film. Application of strain, ε yy , along the viewing direction results in an out-of-plane elastic strain, ε zz , of [33] where ε xx is the in-plane coherency strain that remains unchanged in the clamped film with application of strain along the viewing direction, and c 11 and c 12 are the elastic stiffness constants of the cubic parent material used as reference in the model. At higher compressive ε yy strains the strain ε zz is increased, which results in increased tetragonality of the system and stability of the c -domain [33] , [34] . This leads to the observed switching behaviour of the ferroelastic domain. In contrast, if the indenter is comparable in length scale to the thin film and the film is assumed to be unclamped, the switching behaviour is reversed as shown in Supplementary Fig. 1 . These results are discussed in the Supplementary Discussion . In-plane compression perpendicular to the TEM-viewing direction similarly destabilized the a -domain, as shown in Fig. 6a , which depicts the evolution of partial a -domains along the [100] direction. With increasing compression, the contrast associated with the a -domains changes, ultimately disappears and remains absent on relaxation. The mechanism by which this stress erases the a -domains is straightforward, as compression favours the smaller in-plane lattice parameter of the c -orientation, illustrated in Fig. 6b . Phase-field simulations, shown in Fig. 6c , indicate the a -domains should become progressively and uniformly thinner with increasing strain, and finally vanish at a strain of approximately −0.45%. Together, mechanical switching using both in situ TEM and phase-field simulations show partial ferroelastic domains in the system are highly mobile under all uniaxial loading directions. 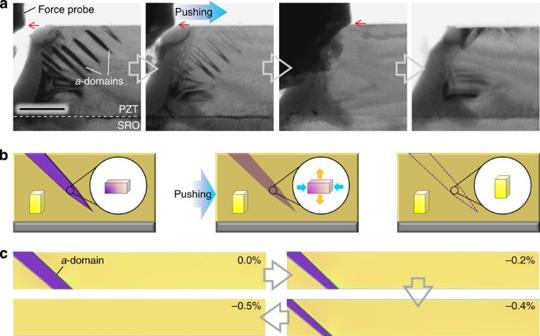Figure 6: Mechanical erasure of ferroelastic domains. (a) Consecutive images showing in-plane stress induced ferroelastic domain erasure. Scale bar, 100 nm. A blunt tip presses the film laterally from the left side and the force is mainly along thexdirection. Domain contrast changes slightly owing to contact stress, eventually disappears and does not come back after removing the probe. The red arrows indicate the induced strain is essentially along the in-plane direction. (b) Schematic showing that the stress favoursc-domain formation and suppresses thea-domain, causing erasure ofa-domains. Left, before contact; middle, squeezing thea-domain; right, thea-domain has been switched to ac-domain. (c) The sequential cross-section plots of domain structures of PZT calculated by phase-field modelling. The extra strainεxxapplied along thexdirection, ranges from −0.2 to −0.5%. The purple colour represents thea-domain, and yellow indicatesc-domain. Thea-domain shrinks and finally disappears with the increasing shear stress. The critical applied strain required to erase ana-domain is about −0.45%. Figure 6: Mechanical erasure of ferroelastic domains. ( a ) Consecutive images showing in-plane stress induced ferroelastic domain erasure. Scale bar, 100 nm. A blunt tip presses the film laterally from the left side and the force is mainly along the x direction. Domain contrast changes slightly owing to contact stress, eventually disappears and does not come back after removing the probe. The red arrows indicate the induced strain is essentially along the in-plane direction. ( b ) Schematic showing that the stress favours c -domain formation and suppresses the a -domain, causing erasure of a -domains. Left, before contact; middle, squeezing the a -domain; right, the a -domain has been switched to a c -domain. ( c ) The sequential cross-section plots of domain structures of PZT calculated by phase-field modelling. The extra strain ε xx applied along the x direction, ranges from −0.2 to −0.5%. The purple colour represents the a -domain, and yellow indicates c -domain. The a -domain shrinks and finally disappears with the increasing shear stress. The critical applied strain required to erase an a -domain is about −0.45%. Full size image In conclusion, the mobility of ferroelastic domains under applied electrical field and mechanical stress is demonstrated by direct observations in TEM in combination with phase-field modelling. The behaviour of the a -domains in response to external excitations is distinctive and is based on their microstructure and configurations within the film. For both sources of stimuli, partial a -domains sitting at free surfaces are always more mobile than those that extend to the bottom interface, which are subject to interface clamping. Dislocations at the substrate interface strongly pin a -domains. Further, through-film a -domains are usually immobile, while a partial a -domain originating at the bottom interface cannot be erased completely by an electric field but can be reversibly extended upwards to the surface of the film through the application of compression at the surface of the film. These results may help explain past disagreements regarding the mobility or immobility of ferroelastic domains, as it depends on which type of ferroelastic domain was present in the area under study. Our results also show that, in ferroelastic needle domains, switching initiates at the high-energy ‘point’ of the needle, where the onset of polarization rotation is observed. One approach to increase the electromechanical response through such switching, therefore, might be to deliberately apply electrical field [16] or strain gradients through mismatch, island patterning, dopant gradients and so on to ensure these ferroelastic domain tips are readily available. Our direct observations that the domain microstructure determines polarization switching characteristics provide new insights into fundamental physics of ferroelectrics and that underpin engineering of nanoscale ferroelectric devices that may include only one or a very few defects in a single cell. Although the observations of switching behaviour are based on the foil geometry of cross-sectional TEM samples, our conclusions can be reasonably assumed to also apply to extended ferroelectric thin film devices owing to the close agreement with the modelling we observed; because the modelling assumes periodic boundary condition along the TEM-viewing direction, no surface effects occur in the model. This implies there is nearly no impact on our results owing to surface effects caused by the foil thinness and are probably unaffected by foil geometry. Furthermore, local switching of ferroelastic domains shown here indicates the possibility of controlling multiple parameters coupled to ferroelastic order in low-symmetry materials, as well as the ability to probe the microstructure dependence of such couplings. Materials synthesis and characterization Tetragonal Pb(Zr 0.2 Ti 0.8 )O 3 (PZT) films oriented in the [001] direction and with ~200 nm in thickness were grown on (001) SrTiO 3 or (110) DyScO 3 substrates buffered by a SRO-conducting electrode with a thickness of 20–50 nm. Cross-sectional TEM specimens were prepared by mechanical polishing followed by argon ion milling (Precision Ion Polishing System, Gatan). In situ TEM experiments were carried out using JEOL 2010F microscope operated at 200 kV in TEM mode equipped with a Nanofactory scanning tunnelling microscopy system at the University of Michigan, and JEOL 3011 microscope operated at 300 kV in TEM mode equipped with a Hysitron nanoindentation system in the Lawrence Berkeley National Laboratory. For electrical switching, a bias voltage was applied between an electrochemically etched tungsten tip, serving as a top electrode, and the conductive SRO bottom electrode that was connected to the holder ground. External voltages were applied using an HP 6614C power supply for direct current voltages. For mechanical indentation, a diamond punch was used. For mechanical erasure of ferroelastic domain, a blunt tungsten tip driven by Nanofactory system was employed to apply in-plane pressure. The evolution of domain structure was imaged in real time using diffraction contrast imaging (diffraction g =(200)) and recorded by a charge-coupled device (Gatan) in JEOL 2010F or television-rate camera (Gatan) in JEOL 3011. High-resolution HAADF-STEM images used in this work were obtained from probe C S -corrected FEI Titan (TEAM 0.5 in Lawrence Berkeley National Laboratory) operating at 300 kV with a semi-convergence angle of 17 mrad, collection angles of [53; 270] mrad and beam current of~0.07 nA. High-resolution STEM image analysis All high-resolution STEM images used for polarization mapping in this work were filtered in Fourier space using a grid mask to select for the lattice frequencies and by low- and high-pass annular filters to remove the zero-frequency and high-frequency noise above the information transfer limit. Atom positions were determined by simultaneously fitting two-dimensional Gaussian peaks to an a priori perovskite unit cell using a home-developed code running in MatLab R2011a. Polar displacements of the Pb cations were measured relative to the centre of the surrounding Zr/Ti cations in HAADF STEM images. Geometric phase analysis was performed using a free FRWRtools plugin for Digital Micrograph by Koch [35] based on the original work by Hytch et al. [36] , [37] The detailed parameters are shown in Supplementary Fig. 2 . Phase-field modelling Ferroelastic switching in the thin film was simulated using the phase-field method by solving the time-dependent Ginzburg–Landau equation for the temporal evolution of the polarization vector field [33] , [34] where P i is the polarization, L is a kinetic coefficient related to the domain wall mobility and F is the volume integral of the system energy that includes contributions from the Landau, elastic and gradient energies. Detailed descriptions of the energy functional F are presented in some depth in our previous publication [33] . This equation was solved by a semi-implicit Fourier spectral method using a discreet grid of 256 Δ x × 1 Δ x × 150 Δ x (Δ x is the number of grid points) with periodic boundary conditions along the x 1 and x 2 axes in the film plane [34] . A thin film was simulated by applying appropriate boundary conditions in the out-of-plane x 3 direction as described in detail in our previous publications [34] , [38] . The spacing of the grid, Δ x , was taken to be 0.5 nm. A thickness of 80 Δ x was used for the film, and a thickness of 40 Δ x was used for the substrate layer that was allowed to mechanically relax. To simulate the thin film, we set a small initial polarization in the out-of-plane direction and allowed the film to relax. By incorporating dislocations as described in the paper, the films were found to relax to include partial ferroelastic domains. Each dislocation was incorporated into the model by explicitly considering the eigenstrains associated with the missing half-plane of atoms between the dislocation core and the free surface of the thin film following the work of Hu [39] and Wang [40] . These eigenstrains were incorporated into the solution for mechanical equilibrium in the system. Mixed elastic boundary conditions were used where the displacement at the bottom of the substrate was assumed to be zero, and the out-of-plane components of the stress were assumed to be zero at the film-free surface [34] . The average residual strain in the thin film was chosen to be −2.1% for the mechanical switching simulations and –1.7% for the electric switching simulations [34] . After equilibrium was reached with a traction-free top surface, mechanical switching was simulated by altering to boundary condition at the free surface of the film to apply a finite σ 33 stress at the film surface. The mechanical indenter was simulated as a rigid cylindrical punch with a bottom surface profile of a 12th-order polynomial to represent a nearly flat bottom that caused an additional displacement, δ , at the top surface of [41] where b is a fitting constant, a is the radius of the punch and r is the distance between a point on the surface of the film and the centre of the cylindrical punch. Throughout the simulations, the indenter was assumed to have a radius of 40 nm. Determining the total load and stress distribution caused by this displacement are described in ref. 41 . The fitting parameter, b , was chosen such that the total load applied by the indenter was as indicated in the main text. Similarly, boundary conditions for the electric equations employed fixed electrical potential at the top and bottom surfaces of the thin film. Potential at the top and bottom surfaces was set to zero to allow the film to reach equilibrium and for the mechanical switching simulations. To simulate switching with an applied electrical potential, the top surface of the film was assumed to be traction free while the potential, φ , at the top surface of the film was set to [42] where φ 0 is the applied potential, γ is the half-width of the electrode and ( x 0 , y 0 ) is the position of the electrode. In this simulation we used an isotropic dielectric constant of ε r =10. The Landau, stiffness and electrostrictive constants used are listed in ref. 34 . How to cite this article: Gao, P. et al. Ferroelastic domain switching dynamics under electrical and mechanical excitations. Nat. Commun. 5:3801 doi: 10.1038/ncomms4801 (2014).